Cementing proteins provide extra mechanical stabilization to viral cages The study of virus shell stability is key not only for gaining insights into viral biological cycles but also for using viral capsids in materials science. The strength of viral particles depends profoundly on their structural changes occurring during maturation, whose final step often requires the specific binding of ‘decoration’ proteins (such as gpD in bacteriophage lambda) to the viral shell. Here we characterize the mechanical stability of gpD-free and gpD-decorated bacteriophage lambda capsids. The incorporation of gpD into the lambda shell imparts a major mechanical reinforcement that resists punctual deformations. We further interrogate lambda particle stability with molecular fatigue experiments that resemble the sub-lethal Brownian collisions of virus shells with macromolecules in crowded environments. Decorated particles are especially robust against collisions of a few k B T (where k B is the Boltzmann’s constant and T is the temperature ~300 K), which approximate those anticipated from molecular insults in the environment. A fundamental intermediate in the development pathway of many double-stranded DNA (dsDNA) viral particles is a procapsid shell into which the genome is packaged. Procapsid intermediates are observed in both bacteriophage and eukaryotic viruses such as adenovirus and the herpesviruses [1] , [2] . Procapsids are typically constructed of a few quasiequivalent proteins that self-assemble into an icosahedral shell aided by a scaffolding protein [3] , [4] , [5] . The portal complex is assembled at a unique vertex to provide a canal for DNA entry and release during packing and infection, respectively [6] . DNA packaging triggers a major re-organization of the proteins assembled into the procapsid. This maturation process, which is essential for generating infectious particles, results in a thinning and increased angularization of the viral shell achieving a structure with enlarged internal volume [7] . Subsequently, the structural integrity of the shell is enhanced using different strategies including: (i) enhanced interactions between the shell proteins [7] ; (ii) autocatalytic covalent crosslinking the shell proteins [8] , [9] , [10] ; or (iii) specific binding of ‘cementing decoration proteins’ to the exterior of the expanded capsid lattice. Bacteriophage lambda, whose developmental pathway is prototypical of eukaryotic herpesviruses and many bacteriophages, adopts the latter approach. The variation of the virus shell stability is concomitant to the structural changes induced by maturation [11] , [12] . Atomic force microscopy (AFM) has been used to define the mechanical properties of individual viruses, and the results of these studies have been interpreted as a signature of capsid shell stability along the maturation pathway [13] , [14] , [15] . In general, while capsid expansion is not accompanied by a noticeable stiffening of the viral shell, the packed genetic material induces a major reinforcement of the virion [16] , [17] , [18] . However, there is a lack of knowledge about the ultimate physical features that allow cementing decoration proteins to stabilize viral capsids as required for survival in crowded environments. Bacteriophage lambda is one of the most studied and characterized dsDNA bacteriophages. The capsid assembly pathway initiates with the self-association of the portal protein gpB into a dodecameric ring structure. This nucleates the assembly of 405 copies of major protein gpE, into an icosahedral shell with a T =7 triangulation number, chaperoned by the gpNu3 scaffolding protein. Upon packaging ~15 kb of DNA, the shell undergoes an expansion transition that exposes hydrophobic surface area to which the gpD cementing protein adds [19] , [20] . The immature capsid is 4 nm thick and 50 nm in diameter, whereas the mature capsid is thin (2 nm) and presents an angularized icosahedral shape of ~65 nm in diameter that can accommodate the 48.5 kbp dsDNA genome. Prior work has demonstrated that procapsid expansion occurs without any processing of the major capsid protein and can be triggered by treatment with urea in vitro . Subsequently, gpD protein adds to hydrophobic patches at the external surface of the expanded shell [21] . While not required for DNA packaging per se , gpD decoration is required to package the full genome length, presumably owing to instability of the shell in its absence. These observations suggest that gpD protein provides the necessary stability to the shell for withstanding the tremendous internal pressure built up during dsDNA packing [22] . In addition, while expanded shells appear fragile under the typical electron microscopy staining preparations, gpD-decorated particles preserve its integrity [21] . These observations have been interpreted to indicate that gpD provides structural stability to the expanded shell, but an objective and systematic demonstration has never been performed on this or any other viral decoration protein. Here we investigate a variety of mechanical properties of each lambda capsid maturation intermediate, including the procapsid, the expanded capsid and the gpD-decorated capsid. Besides the typical single-indentation assays probing virus elasticity and yield force, our methodology also include molecular fatigue experiments that explore the stability of bacteriophage shells to stresses that approximate molecular insults in the environment. We found that the addition of gpD decoration protein to the shell of bacteriophage lambda provides significant mechanical stability. Imaging individual lambda particles To characterize the mechanical properties of the lambda shell intermediates along the maturation pathway ( Fig. 1a ), we have performed nanoindentation experiments using AFM (see Methods section for details). The first step is the correct identification of the viral shells absorbed on HOPG (highly oriented pyrolytic graphite) substrates. High-resolution AFM topographies of viral particles show distinguishable characteristics of the procapsid and capsid structures, such as the hexamers and the vertex pentamers, that correspond to the fivefold symmetry axes ( Fig. 1b,c ). Interestingly, the addition of gpD protein blurs the capsomers, resulting in a less granular appearance of decorated capsids ( Fig. 1d ). The profile topographies of the particles ( Fig. 2 ) are consistent with the dimensions previously obtained by cryo-electron microscopy [19] , [20] , indicating that the particles are not significantly affected by the interaction with the HOPG surface upon adsorption. 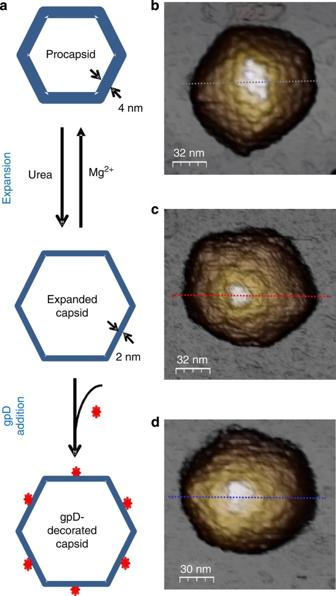Figure 1: Maturation of bacteriophage lambda procapsid. (a) Scheme of structural changes produced during the bacteriophage lambda procapsid maturation. (b–d) High-resolution AFM images of viral particles of bacteriophage lambda absorbed on HOPG: (b) procapsid, (c) expanded capsid and (d) gpD-decorated expanded capsid. Figure 1: Maturation of bacteriophage lambda procapsid. ( a ) Scheme of structural changes produced during the bacteriophage lambda procapsid maturation. ( b – d ) High-resolution AFM images of viral particles of bacteriophage lambda absorbed on HOPG: ( b ) procapsid, ( c ) expanded capsid and ( d ) gpD-decorated expanded capsid. 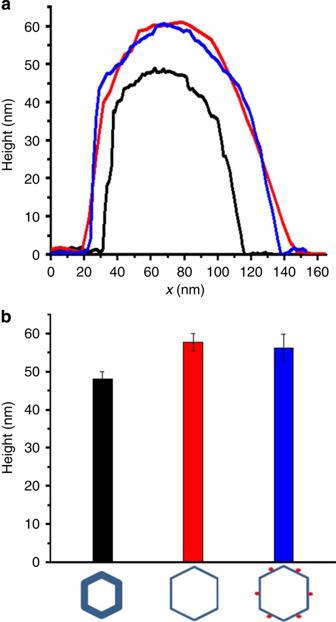Figure 2: Height distribution of viral particles. (a) Height profile along the three kind of viral particles ofFig. 1: procapsid (grey), expanded capsid (red) and gpD-decorated capsid (blue). (b) Column bar representation of the height (mean±s.d.) of 49 procapsids (black), 25 expanded capsids (red) and 30 gpD-decorated capsids (blue). Full size image Figure 2: Height distribution of viral particles. ( a ) Height profile along the three kind of viral particles of Fig. 1 : procapsid (grey), expanded capsid (red) and gpD-decorated capsid (blue). ( b ) Column bar representation of the height (mean ± s.d.) of 49 procapsids (black), 25 expanded capsids (red) and 30 gpD-decorated capsids (blue). Full size image Single-indentation assay In order to study the mechanical properties of the lambda particles, we first implemented a single-indentation assay, consisting in large indentations on multiple viral particles that induce the shell demolition. The resulting force versus indentation curve provides information about the elasticity and yield force of the particles [23] , [24] . In addition, the spring constant/rigidity of each particle is determined from the slope of the linear part of the curve. 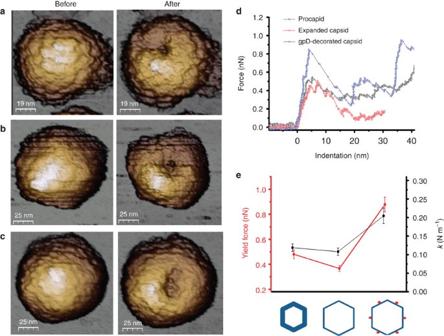Figure 3: Stiffness and yield force. Single-indentation assays performed on viral particles. (a) AFM images of a procapsid, before and after fracture. (b) Same description to expanded capsid. (c) Same description to gpD-decorated capsid. (d) Comparison of nanoindentation curves performed on each particle. (e) Representation of the yield force and stiffness (mean±s.e.) of 16 procapsids, 15 expanded capsids and 15 gpD-decorated capsids. Figure 3 shows the typical evolution of viral shells upon indentation experiments. The force versus distance curve ( Fig. 3d , black) performed on a procapsid ( Fig. 3a , before) induces a crack large enough to collapse the structure ( Fig. 3a , after). It is tempting to assign the force at which the crack is created (yield force) to the elastic limit of the indentation curve (that is, the force value at the first sharp decay after linear indentation). However, the sharp decays of the force can be related to reversible deformations, buckling, slip and rotation of the particle [25] , [26] . Thus, particles were routinely imaged after the indentation experiment and only those showing evident cracking are considered for statistics. Likewise, expanded capsids ( Fig. 3b ) and gpD-decorated capsids ( Fig. 3c ) were also subjected to nanoindentation experiments. In this way, we studied 16 procapsids, 15 expanded capsids and 15 gpD-decorated capsids. The analysis of experimental curves shows that while the procapsid and expanded capsid particles present a similar spring constant (0.12±0.01 N m −1 ) and (0.11±0.01 N m −1 ), respectively, gpD-decorated capsids possess double the stiffness (0.20±0.02 N m −1 ) relative to the non-cemented shells ( Fig. 3e ). Interestingly, while procapsid expansion results in a decrease in the yield force from 0.48±0.03 to 0.37±0.02 nN, addition of the cementing protein significantly strengthens the shell to afford a yield force of 0.88±0.07 nN ( Fig. 3e ). Figure 3: Stiffness and yield force. Single-indentation assays performed on viral particles. ( a ) AFM images of a procapsid, before and after fracture. ( b ) Same description to expanded capsid. ( c ) Same description to gpD-decorated capsid. ( d ) Comparison of nanoindentation curves performed on each particle. ( e ) Representation of the yield force and stiffness (mean ± s.e.) of 16 procapsids, 15 expanded capsids and 15 gpD-decorated capsids. Full size image Molecular fatigue assay In order to complement the single-indentation assay studies and obtain the full picture of the viral shell mechanics, we conducted a second experimental approach based on repeated load experiments [27] . It is known that virus particles exposed to a cyclic load at low forces induces an stepwise disassembly of the individual capsomers of the viral shell [28] . Quantification of the number of load cycles at certain force needed to produce the first damage of the shell structure informs about the stability of single capsomers. Imaging of individual viruses with AFM in jumping plus [29] requires thousands of load cycles at low force ( Fig. 4 ). Therefore, the continuous imaging of a viral particle enables the evaluation of any structural alteration while subjected to cycle load at low forces. Thus, we performed such a study with the lambda capsid intermediates. Figure 5a shows a typical molecular fatigue experiment performed on a single procapsid at 100 pN of force. 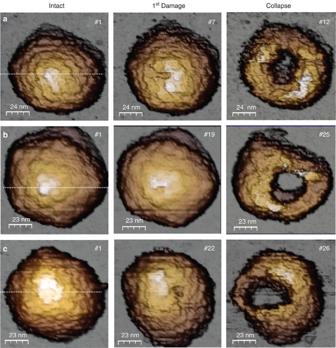Figure 5: Stability under molecular fatigue. Selected topography image frames of viral particles under molecular fatigue experiments: (a) on procapsid (100 pN), (b) expanded capsid (100 pN) and (c) gpD-decorated expanded capsid (120 pN). Labels refer to the ‘#’ of frame within theSupplementary Movies 1, 2 and 3, corresponding to the first damage (central column) and the final collapse (right column). We have selected the frames corresponding to unaltered, fist damage and collapsed particle ( Supplementary Movie 1 ). Shell damage, consisting of capsomer vacants, was first observed at the sixth consecutive image and the shell was fully collapsed at image no. 12. Figure 5b,c present similar experiments on an expanded capsid and a cemented particle at 100 and 120 pN, respectively, ( Supplementary Movies 2 and 3 ). We have detected a common qualitative behaviour: first, a capsomeric vacant appears as a result of molecular fatigue. Subsequently, this vacant induces a crack that further extends throughout the shell until the particle undergoes the total collapse. The evolution along time of the particle topographic profile helps to extract important information. Specifically, the kymographs of the movies obtained along the dashed white lines of Fig. 5 #1 frames, depicted in Fig. 6a , already show some interesting features for each type of particle. For instance, the height evolution obtained at the top of each particle (dashed lines, Fig. 6a ) reveal that at a load force of 100 pN, gpD-decorated particles resist AFM scanning for >5 h (~100 frames) without suffering any damage (blue open circles, Fig. 6b and Supplementary Movie 4 ). In contrast, the procapsid and the expanded capsid demonstrate evident signs of destruction after 6 and 19 frames, respectively. To further probe cemented capsid stability, we increased the force of the load cycles performed on gpD-decorated particles from 100 to 120 pN in order to accelerate the destruction process (blue solid circles, Fig. 6b ). Thus, we performed molecular fatigue experiments on seven procapsids, seven expanded capsids and eight decorated capsids. 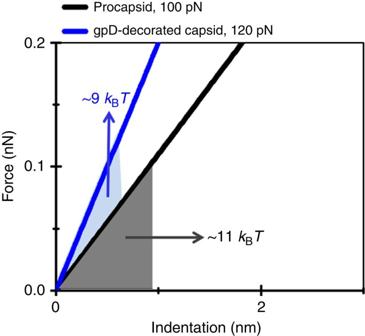Figure 6c shows the average number of cycles (that is, lifetime) needed for inducing the first failure for each kind of particle: while gpD-decorated particles withstand ~1.8 × 10 5 cycles at 120 pN, expanded capsids and procapsids resist for 1.1 × 10 5 cycles at 100 pN and 0.4 × 10 5 cycles at 100 pN, respectively. 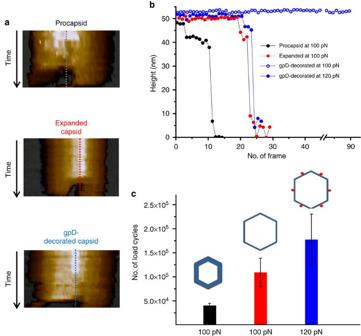Figure 6: Lifetime of viral shells under fatigue. (a) Kymographs of the white lines of profiles in frames no. 1 ofFig. 5. (b) Comparison of the height evolution along time of procapsid (black, 100 pN), expanded capsid (red, 100 pN) and gpD-decorated capsid (solid blue circle, 120 pN). The gpD-decorated capsid remains unaltered under 100 pN (open blue circle,Supplementary Movie 4). (c) Histogram of number of load cycles performed on seven procapsids (black), seven expanded capsids (red) and eight gpD-decorated capsids (blue) to damage the particle (mean±s.e.). Figure 4: Energetics of molecular fatigue. Estimation of the energy per cycle that is supplied to procapsid (dark) and gpD-decorated capsid (blue). Figure 4: Energetics of molecular fatigue. Estimation of the energy per cycle that is supplied to procapsid (dark) and gpD-decorated capsid (blue). Full size image Figure 5: Stability under molecular fatigue. Selected topography image frames of viral particles under molecular fatigue experiments: ( a ) on procapsid (100 pN), ( b ) expanded capsid (100 pN) and ( c ) gpD-decorated expanded capsid (120 pN). Labels refer to the ‘#’ of frame within the Supplementary Movies 1, 2 and 3 , corresponding to the first damage (central column) and the final collapse (right column). Full size image Figure 6: Lifetime of viral shells under fatigue. ( a ) Kymographs of the white lines of profiles in frames no. 1 of Fig. 5 . ( b ) Comparison of the height evolution along time of procapsid (black, 100 pN), expanded capsid (red, 100 pN) and gpD-decorated capsid (solid blue circle, 120 pN). The gpD-decorated capsid remains unaltered under 100 pN (open blue circle, Supplementary Movie 4 ). ( c ) Histogram of number of load cycles performed on seven procapsids (black), seven expanded capsids (red) and eight gpD-decorated capsids (blue) to damage the particle (mean ± s.e.). Full size image Capsid assembly and maturation are highly conserved processes that prepare viruses for infectivity. In the case of the complex dsDNA viruses, the genome is packaged into a pre-assembled procapsid that triggers a series of maturation steps. The latter process involves significant conformational changes in the proteins assembled into the shell, often leading to a remarkable procapsid expansion transition for many viruses. The expansion is followed by the shell stabilization using three basic mechanisms: in some such as HK97 procapsid expansion is accompanied by the formation of a network of covalent crosslinks [10] , [30] , [31] . Others, typified by bacteriophage T7 (ref. 7 ), increase the interaction areas between protein subunits in the expanded shell. Yet other viruses such as bacteriophages T4 (ref. 32 ) and lambda [19] , and the eukaryotic herpesviruses incorporate accessory proteins into the shell. In the case of bacteriophage lambda, the maturation process comprises three distinct shell structures: procapsid, expanded capsid and gpD-decorated capsid ( Fig. 1a ). The evolution of the stiffness and the yield force from procapsids to expanded capsids ( Fig. 3e ) indicates that the shell loses some strength during expansion. Although thin shell modelling [23] applied to lambda geometry would assign to expanded capsids a Young modulus ~5 times larger than procapsids [14] , it is known that the expanded shell is fragile and easily damaged by Transmission electron microscopy (TEM) staining procedures [21] . This finding, together with our results, suggest that the objective of the expansion transition is not the immediate stabilization, as it appears for other phages [30] . For instance, the expanded structures of HK97 show an increment of the yield force with respect the prohead due to the crosslinking [14] . Our results are compatible with the unique observation that expansion of the lambda procapsid is fully reversible [21] , since the capsid contraction would be more difficult with a stiffer particle. Therefore, we can conclude that the main objective of the expansion, besides increasing the shell volume for DNA accommodation, is the exposure of the hydrophobic patches to provide nucleation sites for gpD trimer spike assembly [21] and not the immediate stabilization. Likewise, our experiments demonstrate that gpD incorporation into the shell induces a major mechanical reinforcement of the capsid in both the stiffness and yield force ( Fig. 3e ). This result is again compatible with the previous observation that gpD stabilizes the expanded particles in TEM preparations [21] and with the strict requirement for gpD in viral genome packaging. Although the gpD protein is not required for DNA translocation into the capsid, it is essential for the packaging of the penultimate 8–10 kbp of the viral genome [22] . This finding has been interpreted to indicate that gpD provides to the capsid sufficient structural stability to support the tens of atmospheres internal pressure generated by the packed dsDNA [19] , [20] . Structural data indicate that gpD monomers assemble as a trimer spike at the threefold axes of the expanded shell. The N-terminal tail of each monomer provides a β-strand to complete a four-stranded β-sheet formed by gpD and two adjacent major capsid protein (gpE) monomers in the shell. This is recapitulated 420 times across the surface of the capsid that has been postulated to provide significant structural stabilization to the expanded shell [19] . Our results clearly demonstrate that gpD trimers impart mechanical stability to the shell since the decorated capsids possess an almost doubled spring constant and yield force values relative to both the procapsid and expanded capsid particles. Within this context, it is of interest to compare the mechanical stability provided by gpD in bacteriophage lambda with that obtained by chemical crosslinking in the HK97 capsid. The symmetric disposition of gpD on the capsid surface affords a network of non-covalent interactions that closely mimic those observed in the covalent chemical crosslinked ‘chain-mail’ lattice observed in the mature HK97 shell. However, while covalent crosslinking results in an increase in the yield force of the shell [14] , the stiffness does not increase as we observed in lambda. Overall, we can conclude that the multitude of non-covalent interactions of the cementing protein with the capsid shell are just as effective in mechanically stabilizing viral cages as is physicochemical crosslinking such as observed in HK97. It is noteworthy to mention that we utilized purified procapsid shells that were expanded in vitro and decorated with purified gpD in a rigorously defined reaction mixture [33] . The decorated capsids are fully functional in genome packaging reactions and thus reflect biologically relevant structures. We note that an earlier AFM study utilized ‘phage ghosts’ that are obtained from infectious phage subsequent to genome ejection from the gpD-decorated capsid shell [17] . The prior study reported a lower spring constant than that obtained here, which may reflect subtle modification of the shell resulting from DNA packaging and/or DNA ejection, alteration of the gpD-capsid protein contacts subsequent to DNA ejection, and/or the presence of a finishing proteins and a tail bound to the portal complex. Alternatively, the large tail structure could affect the anchorage stability during particle indentation, thus influencing the mechanical measurements. While the yield force describes the maximal insult survivable by the shell, a viral capsid must also survive a constant barrage of sub-lethal collisions in the environment. Molecular fatigue experiments provide additional mechanical information by reporting on shell stability against such multiple small deformations at low force (~100 pN), well below the yield force ( Fig. 3e ). Consecutive load cycles probe the resilience of inter-capsomer bonds at a local scale, in contrast with the global response obtained with the single-indentation assay. Load cycles mimic the impacts between macromolecules and the virus shell, which strongly depend on the molecular crowding of the media. We may use viscosity η as an indirect parameter for evaluating molecular crowding. Specifically, by knowing the diffusion coefficient D of GFP in the Escherichia coli cytoplasm (5 μm 2 s −1 ; ref. 34 ; T =300 K) and the Stokes radius of GFP R =2.82 nm (ref. 35 ); we can use the Einstein relation for estimating , 15 times larger than water. To make the case, let us consider the bacteria living in the gut, where the viscosity of the environment (chyle) is about η ext =1 poise (ref. 36 ), ~7 η host . Therefore, mature capsids immersed in the chyle withstand a higher molecular crowding than inside of the bacterial cytoplasm. This crowding generates continuous impacts between molecules and viral shells with an average energy of 3/2 k B T , where k B is the Boltzmann’s constant and T ~300 K. Interestingly, the energy provided to the viral particles by the tip during each load cycle is ~10 k B T ( Fig. 4 ). Thus, our molecular fatigue experiments can be considered as an accelerated bench test, where viral shells are subjected to the tip impacts, mimicking those of macromolecules in the environment. Our studies show a monotonic stabilization of lambda phage structures along maturation against cycle load ( Fig. 6c ), with gpD incorporation to the capsid providing the major stability to the particles (open blue circle, Fig. 6b ). We increased the fatigue force ~20% in order to induce a minimum structural damage (solid blue circle, Fig. 6b ), and yet strikingly the gpD-decorated particles surpass the lifetime of capsids and procapsids under these stringent conditions ( Figure 6c ). In addition, it is interesting to highlight that while cycle load experiments reveal that the expanded capsid is more stable than procapsid, its spring constant and yield force are slightly lower. This result suggests that expanded capsids would endure longer than proheads against the molecular collisions of a crowded environment. We have studied the mechanical stability of bacteriophage lambda capsid intermediates along the maturation pathway using single-indentation and molecular fatigue assays. From individual indentations, we have found that, while the expanded capsids possess a slightly decreased stiffness and yield force, gpD addition to the expanded shell provides a significant increase (double) in both values. Likewise, our molecular fatigue studies unveil a monotonic increment of stability along the maturations pathway, although once again gpD decoration induces the major stabilization. Our data demonstrate that gpD addition to the shell provides mechanical reinforcement such that the capsid can withstand not only internal stress generated by the tightly packaged genome but also from external physical stress. We show that non-covalent addition of a decoration protein to the capsid shell provides significant mechanical stability to the structure that rivals that observed by covalent chemical crosslinking of the shell proteins. Expression and purification of bacteriophage lambda procapsid Two liters of 2X-YT media, pH 7.2, containing 25 mM potassium phosphate, 5 mM glucose, and 50 μg ml −1 ampicillin was inoculated with a 20-ml overnight culture of E. coli BL21(DE3)[pLysS][pT7Cap] [37] cells derived from an isolated colony. The culture was maintained at 37 °C until an OD 650 of 0.6–0.7 was obtained at which point IPTG (Isopropyl β-D-1-thiogalactopyranoside) was added to a final concentration of 0.5 mM. The incubation was continued for additional 2 h and the cells were harvested by centrifugation. Unless otherwise indicated, all subsequent steps were performed at 0–4 °C. The cell pellet was resuspended in 50 ml ice-cold TMS buffer (50 mM Tris–HCl, pH 8.0, containing 20 mM MgCl 2 and 100 mM NaCl), the cells were lysed by French Press (10,000 psi), and the crude lysate was clarified by centrifugation (7,650 g , 25 min). The procapsids were then harvested by centrifugation (87,200 g, 3h) and the pellets were overlaid with 1 ml TMS buffer and left at 4 °C overnight. The buffer was removed from each tube and the combined extracts were loaded onto a 5-ml HiTrap Q Sepharose High Performance strong anion exchange column (GE Healthcare Life Sciences) equilibrated with TM buffer (50 mM Tris–HCl, pH 8.0, containing 20 mM MgCl 2 ). The column was developed with a 10–500-mM NaCl gradient, and procapsid-containing fractions were pooled, dialysed against TM buffer and concentrated using a 100-kDa MWCO centrifugal filter (Amicon). The sample was applied to a 10–40% sucrose gradient in the same buffer that was centrifuged to equilibrium (87,200 g , 3 h), and the procapsid band was visualized in ambient light. The band was harvested by aspiration and dialysed against TM buffer. The procapsids were then concentrated using a 100-kDa MWCO centrifugal filter and stored at 4 °C until use. Preparation of expanded and gpD-decorated capsid shells Expanded capsid shells were prepared as previously described [33] . In brief, purified procapsids (30 nM) were incubated in 10 mM Tris buffer, pH 8, containing 2.5 M urea and 3 mM MgCl 2 for 10 min on ice. Urea was then removed from the sample by buffer exchange using a 100-kDa MWCO centrifugal filter unit (Amicon) to afford a preparation of expanded capsid shells in 10 mM Tris buffer, pH 8, containing less than 0.5 M urea and 0.5 mM MgCl 2 . The viral decoration protein, gpD, was purified by published procedure [33] . In brief, gpD was expressed from BL21(DE3)[pLysS][pT7Cap] cells and was precipitated from the crude cell lysate with ammonium sulphate. GpD in the ammonium sulphate pellet was purified by DEAE (diethylaminoethyl cellulose) and S-300 gel filtration chromatography, as described. To prepare gpD-decorated capsids, purified gpD (20 μM) was added to the expanded shells (30 nM capsids; 16.2 μM major capsid protein) and the mixture was incubated for 30 min at room temperature. The particles were then buffer exchanged using a 100-kDa MWCO centrifugal filter unit (Amicon) to remove any unreacted gpD and to afford gpD-decorated, expanded capsid shells. The procapsids, the expanded capsids and the gpD-decorated capsids all contain a portal complex but are devoid of scaffolding protein and the viral tail structure; importantly, all of the particles are catalytically active in the in vitro genome packaging reaction [33] , [37] . AFM experiments Stocks of viral particles of bacteriophage lambda were stored in TMS buffer (20 mM MgCl 2 and 50 mM Tris, pH 7.8) to procapsids and Tris buffer (50 mM Tris) to expanded capsids and gpD-decorated capsids. A drop of 20 μl stock solution of viral particles was left on HOPG (ZYA quality NTMDT) for 30 min and washed with buffer. The tip was prewetted with 20 μl of corresponding buffer. The AFM (Nanotec Electrónica S.L., Madrid, Spain) was operated in jumping mode in liquid [38] using rectangular cantilevers RC800PSA (Olympus, Tokyo, Japan) with nominal spring constants of 0.05 N m −1 . Cantilevers spring constants were routinely calibrated by using the Sader’s method [39] . To determine the stiffness of procapsid, expanded capsid and decorated capsid, once individual particles were located on the surface, the lateral piezo scan was stopped when the tip was on top of the particle. Then, force versus distance curves were obtained by elongating the z -piezo until the tip established mechanical contact with the viral particle. The viral particle is indented once, at a high enough force to induce shell damage. Following each F versus Z , an image of the virus is taken to confirm that it does not conserve its integrity or present structural damage. The F versus Z speed is ~50 nm s −1 (ref. 40 ). During the first stages of indentation, the viral particles show a linear deformation [41] that provides the spring constant of the virus k v . For performing the molecular fatigue experiments, we recorded 128 × 128 point images of viral particles. We use the lowest force needed to reach high resolution of structure and avoid its mobility [29] (100 pN). Images were processed using the WSxM software [42] . To build the movies of each particle, all the images were aligned to remove the drift effects. How to cite this article: Hernando-Pérez, M. et al. Cementing proteins provide extra mechanical stabilization to viral cages. Nat. Commun. 5:4520 doi: 10.1038/ncomms5520 (2014).